The occurrence of intracranial rhabdoid tumours in mice depends on temporal control ofSmarcb1inactivation Rhabdoid tumours (RTs) are highly aggressive tumours of infancy, frequently localized in the central nervous system (CNS) where they are termed atypical teratoid/rhabdoid tumours (AT/RTs) and characterized by bi-allelic inactivation of the SMARCB1 tumour suppressor gene. In this study, by temporal control of tamoxifen injection in Smarcb1 flox/flox ;Rosa26-Cre ERT2 mice, we explore the phenotypes associated with Smarcb1 inactivation at different developmental stages. Injection before E6, at birth or at 2 months of age recapitulates previously described phenotypes including embryonic lethality, hepatic toxicity or development of T-cell lymphomas, respectively. Injection between E6 and E10 leads to high penetrance tumours, mainly intra-cranial, with short delays (median: 3 months). These tumours demonstrate anatomical, morphological and gene expression profiles consistent with those of human AT/RTs. Moreover, intra- and inter-species comparisons of tumours reveal that human and mouse RTs can be split into different entities that may underline the variety of RT cells of origin. Rhabdoid tumours (RTs) are highly aggressive cancers affecting infants and young children. They occur at various anatomic locations, including kidney, soft parts and the central nervous system (CNS), where they constitute a specific entity termed atypical teratoid rhabdoid tumours (AT/RTs) [1] . Expression profilings suggest stem cells as potential cells of origin for RTs, in keeping with their remarkably early onset [2] , [3] , [4] . The main genetic hallmark of all RTs is their unique genomic stability, and SMARCB1 inactivation is the only recurrent genetic event [5] , [6] . From a clinical point of view, highly intensive treatments are currently evaluated to achieve better survival [7] , but the poor prognosis and the long-term sequels of such intensive treatments in infants remain major causes of concern. Hence, faithful preclinical models are warranted. Attempts to recapitulate RT in murine models have met with variable success. Although homozygous knockout Smarcb1 leads to early embryonic lethality, Smarcb1 heterozygous mice are prone to developing tumours resembling human RTs [8] , [9] , [10] . However, these tumours almost exclusively develop from soft parts of neck with a long latency and a weak penetrance; almost no brain tumour is reported in those models. Conditional inactivation using a Smarcb1 inv ;Mx-Cre model leads to highly aggressive, fully penetrant tumours, which were demonstrated to be CD8(+), mature peripheral T-cell lymphomas [11] . Thus a genuine murine model for RT, and specifically for AT/RT, is still lacking. In this study, we have generated genetically modified mice that allow conditional inactivation of Smarcb1 , by intercrossing Rosa26-Cre ERT2 (ref. 12 ) and Smarcb1 flox/flox mice [13] . Injection of tamoxifen at various time points allows a sequential inactivation of Smarcb1 from early embryonic stages to adulthood. We show that the time for Smarcb1 inactivation dramatically affects the phenotype. Moreover, we show that early embryonic inactivation of Smarcb1 leads to a fully penetrant model of tumours, mainly intra-cranial, which faithfully resemble human RTs and recapitulate some of their diversity. Smarcb1 inactivation in adult mice leads to lymphomas Because the cell of origin of RT is unknown, we chose the ubiquitously active locus Rosa26 to drive Cre ERT2 expression and subsequent Smarcb1 deletion. We first targeted Smarcb1 by tamoxifen injection in adult mice (that is, 8 weeks). In agreement with Hameyer et al . [12] , we found an efficacious recombination in all tested organs except brains ( Fig. 1a ). As a result, we constantly obtained rapidly fatal tumours, massively infiltrating the liver and the spleen, in a median delay of 12 weeks ( Fig. 1b,c ); this phenotype was not observed in any mice treated with vehicle only ( Fig. 1b–d ). Consistently, Baf47 immunostaining was completely negative in the tumour cells, whereas its ubiquitous expression remains intact in normal contiguous cells ( Fig. 1d ) as in normal tissues of control mice ( Fig. 1d ). Smarcb1 negative cell islets were also occasionally found in lungs and kidneys, but we did not observe any tumour in the CNS. 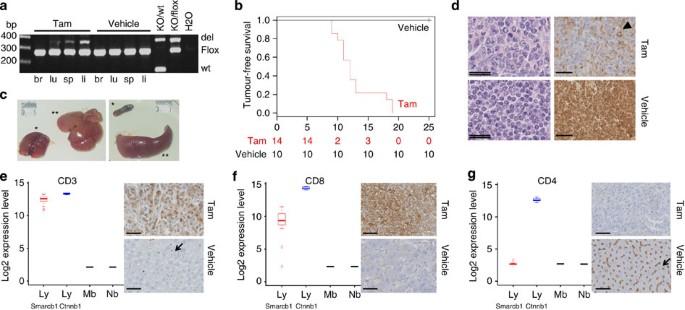Figure 1: Mouse CD8(+) T-cell lymphomas. (a) PCR with primers specifically designed for the deleted (del), the undeleted (flox) and the wild-type (wt) alleles ofSmarcb1in brain (br), lung (lu), spleen (sp) and liver (li); left panel: 5 days after injection of 2 mg per 20 g tamoxifen (Tam); right panel: mouse treated with vehicle. KO/wt: deleted and wild-type alleles from theSmarcb1wt/del_ex2strain. KO/flox: deleted and flox alleles fromSmarcb1del_ex2/floxstrain. (b) Tumour-free survival curve (Kaplan–Meier method) ofSmarcb1flox/flox;Rosa26-CreERT2when tamoxifen (tam) is injected at 8 weeks of age; time in weeks. (c) Macrospcopic aspect of liver (**, left panel) and spleen (**, right panel) inSmarcb1flox/flox;Rosa26-CreERT2mouse when tamoxifen is injected at 8 weeks, as compared with liver and spleen fromSmarcb1flox/flox;Rosa26-CreERT2mouse treated with vehicle (*, left and right panels, respectively). (d) HES (left panels) and BAF47 immunostaining (right panels) on spleen fromSmarcb1flox/flox;Rosa26-CreERT2mouse treated with tamoxifen (upper panel) and vehicle (lower panel); tumour cells and loss of Baf47 expression are observed in tamoxifen treated organs only. The arrows show positive internal controls. Simple scale bars, 50 μm; double scare bars, 25 μm. (e–g) High expression of CD3 (e), high expression of CD8 (f) and low expression of CD4 (g) assessed by Affymetrix MOE430 2.0 arrays (left panels) and immunostaining (right panels). For histological sections, simple scale bars, 50 μm. CD3, CD8 and CD4 immunostainings are shown in livers fromSmarcb1flox/flox;Rosa26-CreERT2treated with tamoxifen (Tam, upper panels) or vehicle (lower panels). Arrows show normal lymphocytes (CD3 positive staining) and Kuppfer cells (CD4 positive staining) in control livers; the normal hepatic architecture is completely abolished in the CD8+/CD4− lymphomas. For Affymetrix data, expression in theSmarcb1-deficient tumours (Lymphsmarcb1,n=7) are compared with medulloblastomas from thePtch1+/−model (Mb,n=4), neuroblastomas from the Th-Mycn model (Nb,n=3), and T-cell lymphomas from theCtnnb1del-ex3model (Lymphctnnb1,n=7). In box plots, the central rectangle spans the first quartile to the third quartile (interquartile range or IQR); the horizontal line inside the rectangle shows the median; whiskers are taken to 1.5 × IQR from the quartile; circles show outliers. Figure 1: Mouse CD8(+) T-cell lymphomas. ( a ) PCR with primers specifically designed for the deleted (del), the undeleted (flox) and the wild-type (wt) alleles of Smarcb1 in brain (br), lung (lu), spleen (sp) and liver (li); left panel: 5 days after injection of 2 mg per 20 g tamoxifen (Tam); right panel: mouse treated with vehicle. KO/wt: deleted and wild-type alleles from the Smarcb1 wt/del_ex2 strain. KO/flox: deleted and flox alleles from Smarcb1 del_ex2/flox strain. ( b ) Tumour-free survival curve (Kaplan–Meier method) of Smarcb1 flox/flox ;Rosa26-Cre ERT2 when tamoxifen (tam) is injected at 8 weeks of age; time in weeks. ( c ) Macrospcopic aspect of liver (**, left panel) and spleen (**, right panel) in Smarcb1 flox/flox ;Rosa26-Cre ERT2 mouse when tamoxifen is injected at 8 weeks, as compared with liver and spleen from Smarcb1 flox/flox ;Rosa26-Cre ERT2 mouse treated with vehicle (*, left and right panels, respectively). ( d ) HES (left panels) and BAF47 immunostaining (right panels) on spleen from Smarcb1 flox/flox ;Rosa26-Cre ERT2 mouse treated with tamoxifen (upper panel) and vehicle (lower panel); tumour cells and loss of Baf47 expression are observed in tamoxifen treated organs only. The arrows show positive internal controls. Simple scale bars, 50 μm; double scare bars, 25 μm. ( e – g ) High expression of CD3 ( e ), high expression of CD8 ( f ) and low expression of CD4 ( g ) assessed by Affymetrix MOE430 2.0 arrays (left panels) and immunostaining (right panels). For histological sections, simple scale bars, 50 μm. CD3, CD8 and CD4 immunostainings are shown in livers from Smarcb1 flox/flox ;Rosa26-Cre ERT2 treated with tamoxifen (Tam, upper panels) or vehicle (lower panels). Arrows show normal lymphocytes (CD3 positive staining) and Kuppfer cells (CD4 positive staining) in control livers; the normal hepatic architecture is completely abolished in the CD8+/CD4− lymphomas. For Affymetrix data, expression in the Smarcb1 -deficient tumours (Lymph smarcb1 , n =7) are compared with medulloblastomas from the Ptch1 +/− model (Mb, n =4), neuroblastomas from the Th-Mycn model (Nb, n =3), and T-cell lymphomas from the Ctnnb1 del-ex3 model (Lymph ctnnb1 , n =7). In box plots, the central rectangle spans the first quartile to the third quartile (interquartile range or IQR); the horizontal line inside the rectangle shows the median; whiskers are taken to 1.5 × IQR from the quartile; circles show outliers. Full size image This phenotype, consisting of aggressive Smarcb1 -deficient malignancy massively involving the spleen and the liver, was very much reminiscent of the mature CD8(+) T-cell lymphomas reported by Roberts et al . in Smarcb1 inv ;Mx1-Cre model [11] . To confirm this similarity, we compared the expression profiles of our tumours with a data set of non- Smarcb1 -deficient tumours profiled on the same Affymetrix MOE430 arrays, consisting of Shh medulloblastomas (Mb, Ptch1 +/− model, provided by O.A.) and neuroblastomas (Nb, Th-Mycn model from our laboratory [14] ); since lymphomas from Roberts’ model were not analysed on the same array, we also aimed to compare our tumours with comparable, still different, lymphomas available from public data sets (CD8(+)CD4(+) lymphomas from ref. 15 ). Welch t -test-based comparisons followed by DAVID and Ingenuity Pathways Analyses highlighted the T-cell-like features of those tumours ( Supplementary Fig. 1 ; Supplementary Data 1 ). More specifically, expression profiling and immunostaining confirmed that they strongly expressed CD3 ( Fig. 1e ) and CD8 ( Fig. 1f ), but did not express CD4 ( Fig. 1g ). Altogether, we concluded that targeting Smarcb1 in adult mice leads to CD8(+)T-cell lymphomas, in full consistency with the CD8(+)T lymphomas previously described. However, as reported by Roberts et al ., this model fails to give rise to any CNS tumour, which could at least be partly explained by a reduced recombination rate induced by Mx1-Cre (10% (ref. 16 )) or Rosa26-Cre ( Fig. 1a and ref. 12 ) in the adult brain. Smarcb1 inactivation in neonates is lethal, without tumour Given the early onset of RTs in humans and the failure to obtain RTs in adult mice, we hypothesized that targeting Smarcb1 earlier in life may better mimic the actual clinical presentation of RTs. This first prompted us to inactivate Smarcb1 in neonates. Semi-quantitative PCR in neonates treated with tamoxifen ( Supplementary Fig. 2a ) showed an actual recombination in all tested organs, including the brain and liver, yet with various efficacies. Smarcb1 inactivation at P2-P3 led to severe growth failure ( Fig. 2a ) and constant rapid death, within the first month ( Fig. 2b ). However, extensive dissection of the mice did not show any tumour. In contrast, microscopic observation of liver sections showed massively vacuolized hepatocytes ( Fig. 2c–h ). In a context of specific hepatic Smarcb1 deletion [13] , Gresh et al . previously reported a dramatically reduced glycogen storage in Smarcb1 -deficient hepatocytes. Thus, we hypothesized that the hepatic phenotype we observed in our model could result from the same metabolic disturbances. Periodic Acid Schiff (PAS) staining confirmed that Smarcb1 -deleted cells actually show reduced glycogen storage as compared with control mice ( Fig. 2c–e,i ). Other organs did not show obvious abnormality. Therefore, we assumed that a major failure in carbohydrate metabolism at least partly explained the death of those mice in short delays, which potentially precluded any tumour to develop. To circumvent this early lethality, we then used half doses of tamoxifen. Mice treated accordingly still showed growth failure and a high rate of death (60%) ( Fig. 2b ), at least partly related to the same, though mildly attenuated, hepatic phenotype ( Fig. 2c–i ). However, the 40% surviving mice did not develop any tumour ( Fig. 2b ). 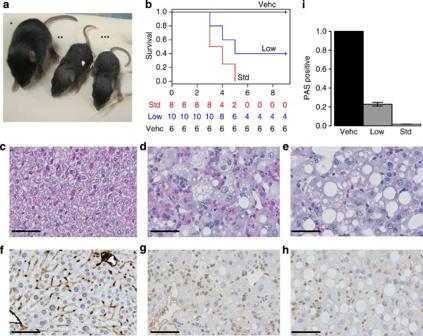Figure 2: Phenotype of neonates uponSmarcb1inactivation. (a) Growth failure of mice treated with low doses (**) (1 mg per 20 g) and standard doses (***) (2 mg per 20 g) as compared with mice treated with vehicle (*) (b) Survival curve (Kaplan–Meier method) of neonates treated with vehicle (black line), low doses (blue line) and standard doses (red line) of tamoxifen. PAS (c–e) and Baf47 (f–h) staining on liver from mice treated with vehicle (c,f), low doses (d,g) and standard doses (e,h) of tamoxifen. (i) Quantification of the PAS staining in mouse treated with vehicle (vehc,n=6), low doses (low,n=6) and standard doses (std,n=6) of tamoxifen. The bars represent the s.e. Scale bars, 50 μm. Figure 2: Phenotype of neonates upon Smarcb1 inactivation. ( a ) Growth failure of mice treated with low doses (**) (1 mg per 20 g) and standard doses (***) (2 mg per 20 g) as compared with mice treated with vehicle (*) ( b ) Survival curve (Kaplan–Meier method) of neonates treated with vehicle (black line), low doses (blue line) and standard doses (red line) of tamoxifen. PAS ( c – e ) and Baf47 ( f – h ) staining on liver from mice treated with vehicle ( c , f ), low doses ( d , g ) and standard doses ( e , h ) of tamoxifen. ( i ) Quantification of the PAS staining in mouse treated with vehicle (vehc, n =6), low doses (low, n =6) and standard doses (std, n =6) of tamoxifen. The bars represent the s.e. Scale bars, 50 μm. Full size image Reduced Smarcb1 deletion prevents embryonic lethality Based again on the early onset of RTs, with occasional antenatal and congenital presentations [17] , we finally postulated that inactivation of Smarcb1 during the embryonic development may actually be relevant to induce RTs in mice. We therefore injected tamoxifen at standard doses (1.5–2 mg per 20 g) in pregnant mice from E1 to E18. In line with the early embryonic lethality of KO models previously reported [8] , [9] , no Smarcb1 deleted pup was obtained when Smarcb1 was inactivated between E1 and E5. When injected between E6 and E10, standard doses of tamoxifen constantly lead to early post-natal lethality of Smarcb1 flox/flox ;Rosa26-Cre ERT2 pups. We assumed that the lethality provoked by standard doses of tamoxifen during the earliest stages of embryonic development was due to an excessive deletion of Smarcb1 , as reported previously [11] . However, we successfully circumvented the lethality provoked at the earliest stages by using lower doses of tamoxifen ( Supplementary Fig. 3 ). As a result, our model allowed us to investigate the phenotypes associated with Smarcb1 inactivation at various developmental stages, from E6 to E18. High penetrance and rapid onset of CNS tumours We administered tamoxifen in pregnant mice from E6 to E18, using reduced doses of tamoxifen from E6 to E12 and normal doses from E12 to E18 ( Supplementary Fig. 3 ). As a result, the fraction of living pups was normal at all stages. By semi-quantitative PCR and using Rosa26-LacZ reporter strain, we first demonstrated that the recombination was ubiquitous at all stages, though in variable degrees ( Supplementary Fig. 2 ). In particular, Smarcb1 locus was recombined in the brain at all stages, but with a higher efficacy before E12 ( Supplementary Fig. 2a,b ). Baf47 immunostaining nevertheless clearly showed Smarcb1 -deficient cells scattered in the CNS without specific anatomical pattern, when tamoxifen was injected at E6, E9 or E12 ( Fig. 3 ). 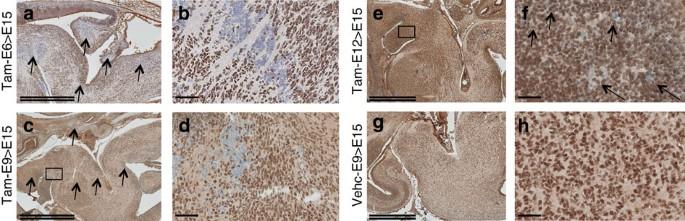Figure 3:Smarcb1-deficient cells at E15 are scattered in the whole CNS. Baf47 immunostaining is performed at E15 on brains (centred on pons and posteriori fossa) from mice treated at (a,b) E6, (c,d) E9 and (e,f) E12 with tamoxifen (1 mg per 20 g); (g,h) control E15 brain after treatment with the vehicle at E9 (same results when the vehicle is injected at E6 and E12). Higher magnifications on the right panels focus on theSmarcb1-deficient cells; arrows depictSmarcb1-deficient areas or cells. Double scale bars, 1 mm; single scale bars, 50 μm. Figure 3: Smarcb1 -deficient cells at E15 are scattered in the whole CNS. Baf47 immunostaining is performed at E15 on brains (centred on pons and posteriori fossa) from mice treated at ( a , b ) E6, ( c , d ) E9 and ( e , f ) E12 with tamoxifen (1 mg per 20 g); ( g , h ) control E15 brain after treatment with the vehicle at E9 (same results when the vehicle is injected at E6 and E12). Higher magnifications on the right panels focus on the Smarcb1 -deficient cells; arrows depict Smarcb1 -deficient areas or cells. Double scale bars, 1 mm; single scale bars, 50 μm. Full size image Strikingly, inactivation of Smarcb1 at E6-E7 almost constantly resulted in intra-cranial (hippocampus region, cerebellum and cerebral cortex) ( Fig. 4a,b ) or spinal tumours ( Fig. 4c ), revealed by neurological defects (gait disturbance or paraplegia), in a median delay of 90 days ( Fig. 4d ). One tumour only arose from a paw, in the soft parts. The tumour penetrance decreased when tamoxifen was administered from E8 to E10 ( Fig. 4d ); it became null from E11 to E18 ( Fig. 4d ). 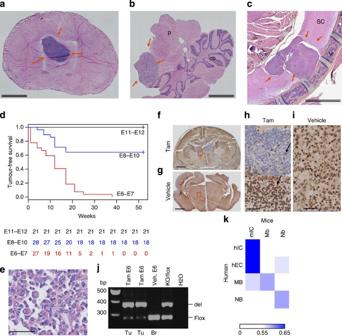Figure 4: Characteristics of mouseSmarcb1-deficient tumours. Macroscopic dissection of the CNS inSmarcb1flox/flox;Rosa26-CreERT2showing tumours. (a) In the sub-ependymal region, (b) in the ponto-cerebellum angle, (cb, cerebellum; p, pons) and (c) in the spinal cord (v, vertebra; sc, spinal cord). Double scale bars, 2 mm. (d) Tumour-free survival after tamoxifen injection (0.5–1 mg per 20 g) at E6–E7, E8–E10 and E11–E12; time in weeks. Numbers are reported under the curve for each category. (e) Rhabdoid phenotype of tumour cells (hematoxylin eosin safran staining): prominent nucleoli, uncondensed nuclei, eosinophilic cytoplasmic inclusions. (f–i) Baf47 immunostaining; low magnification of a coronal section at P2 of brains inSmarcb1flox/flox;Rosa26-CreERT2mice treated at E6 with tamoxifen (Tam) (f) and vehicle (g); higher magnification of the same coronal sections (h,i). Areas with negative staining are seen in mice treated with tamoxifen only; normal internal controls stain positively (arrows). Single scale bars, 50 μm. (j) PCR with primers specifically designed for the deleted (del) and undeleted (flox) alleles ofSmarcb1;Tu, 2 different brain tumours veh, vehicle; KO/flox, control DNA from of aSmarcb1del_ex2/floxmouse; (k) AGDEX correlation score performed on all ortholog genes comparing a set of mouse and human tumours. The reference tissues used for the comparisons were normal cerebral cortex in both species. Matched control tumours: humanSHHmedulloblastomas (MB) and mouse medulloblastomas (Mb,Ptch1+/−model); humanMYCN-amplified neuroblastomas (NB) and mouse neuroblastomas (Nb, Th-Mycn model). Figure 4: Characteristics of mouse Smarcb1- deficient tumours. Macroscopic dissection of the CNS in Smarcb1 flox/flox ;Rosa26-Cre ERT2 showing tumours. ( a ) In the sub-ependymal region, ( b ) in the ponto-cerebellum angle, (cb, cerebellum; p, pons) and ( c ) in the spinal cord (v, vertebra; sc, spinal cord). Double scale bars, 2 mm. ( d ) Tumour-free survival after tamoxifen injection (0.5–1 mg per 20 g) at E6–E7, E8–E10 and E11–E12; time in weeks. Numbers are reported under the curve for each category. ( e ) Rhabdoid phenotype of tumour cells (hematoxylin eosin safran staining): prominent nucleoli, uncondensed nuclei, eosinophilic cytoplasmic inclusions. ( f – i ) Baf47 immunostaining; low magnification of a coronal section at P2 of brains in Smarcb1 flox/flox ;Rosa26-Cre ERT2 mice treated at E6 with tamoxifen (Tam) ( f ) and vehicle ( g ); higher magnification of the same coronal sections ( h , i ). Areas with negative staining are seen in mice treated with tamoxifen only; normal internal controls stain positively (arrows). Single scale bars, 50 μm. ( j ) PCR with primers specifically designed for the deleted (del) and undeleted (flox) alleles of Smarcb1; Tu, 2 different brain tumours veh, vehicle; KO/flox, control DNA from of a Smarcb1 del_ex2/flox mouse; ( k ) AGDEX correlation score performed on all ortholog genes comparing a set of mouse and human tumours. The reference tissues used for the comparisons were normal cerebral cortex in both species. Matched control tumours: human SHH medulloblastomas (MB) and mouse medulloblastomas (Mb, Ptch1 +/− model); human MYCN -amplified neuroblastomas (NB) and mouse neuroblastomas (Nb, Th-Mycn model). Full size image Smarcb1 -deficient mouse tumours resemble human RTs The histological analysis of those tumours showed small round undifferentiated features, resembling human primitive neuro-ectodermal tumour, or cytoplasmic eosinophilic inclusions, uncondensed chromatin and prominent nucleoli, highly suggestive of rhabdoid features ( Fig. 4e ). As expected, all tumours showed a complete loss of Smarcb1 expression, while vehicle-treated brains showed a homogenously positive staining ( Fig. 4f–i ). We confirmed that the loss of Baf47 staining was actually due to a deletion of the floxed allele in all tumours tested ( Fig. 4j ). Hence, histological and genetic patterns were very similar to human RTs. To address the relevance of these mouse tumours for human diseases, we profiled a set of 50 human RTs including 30 intra-cranial (hIC) and 20 extra-cranial (hEC) tumours from various locations (clinical annotation summarized in Supplementary Data 1 ) and compared these expression profiles with those of mouse tumours using AGDEX algorithm designed for cross-species comparison [18] . We first calculated AGDEX scores of human SHH medulloblastomas and MYCN -amplified neuroblastomas with mouse medulloblastomas ( Ptch1 +/− model) and mouse neuroblastomas (Th-Mycn model), respectively. These are two well-established models known to recapitulate their human counterparts: AGDEX scores were 0.58 and 0.59, respectively ( Fig. 4k ). Interestingly, Smarcb1 -deficient intracranial tumours from our model showed even higher AGDEX correlation scores when compared with hIC and hEC (0.67 and 0.68, respectively), confirming their relevance to human RTs ( Fig. 4k ). Diversity within mouse Smarcb1 -deficient tumours To further characterize those mouse tumours, we applied three orthogonal unsupervised clustering methods: unsupervised hierarchical clustering, consensus clustering and non-negative matrix factorization (NMF). We thus compared all Smarcb1- deficient (from Smarcb1 wt/del_ex1-2 and Smarcb1 flox/flox ;Rosa26-Cre ERT2 models, that is, lymphomas, intracranial tumours and extracranial tumours) and non Smarcb1 -deficient mouse tumours aforementioned (medulloblastomas and neuroblastomas). The hierarchical unsupervised clustering ( Supplementary Fig. 4a ) distinguished two main branches (i) the first one consisting of three subgroups made of medulloblastomas, neuroblastomas and a subset of intracranial Smarcb1 -deficient tumours (a group hereafter referred to as mIC), and (ii) the second one consisting of two subgroups, one made of Smarcb1 -deficient lymphomas only, and the last one made of the two extracranial tumours and the remaining intracranial tumours (a group hereafter referred to as mE/IC). Consistently, a Pearson correlation matrix demonstrated that half of the intracranial tumours correlated with extracranial tumours but did not correlate at all with the other half of intracranial tumours ( Supplementary Fig. 4b ). To confirm those results, we next performed NMF ( Supplementary Fig. 4c ) and consensus clustering ( Fig. 5a ; Supplementary Fig. 4d ) on the same data set, Mb and Nb serving as controls for truly existing groups. Thereby, the optimal k value that allows splitting Mb and Nb also defined three tumour groups within Smarcb1 -deficient tumours: CD8(+)T-cell lymphomas and two other subgroups ( Fig. 5a ). One consisted exclusively in intracranial tumours (corresponding to mIC), and the other consisted in the two extracranial tumours and the remaining intracranial tumours (corresponding to mE/IC). Altogether, these results converge to split our intracranial tumours in two distinct entities, one clustering with extracranial Smarcb1 -deficient tumours, and the other clustering close to tumours of neuronal origin, that is, medulloblastomas and neuroblastomas. 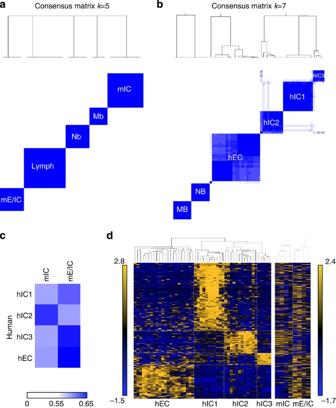Figure 5: Mouse CNS tumours reflect the diversity of human RTs. (a) Differential subgroups were identified using ConsensusClusterPlus R package v1.18.0 (with 1,000 resamplings, average linkage hierarchical clustering algorithm and Pearson correlation distance), based on the expressed and variable genes obtained after elimination of background (threshold: 1.2) and invariant genes using RIQR (threshold: 0.75; max(Q3−Q2,Q1−Q2)/Q2). Mb, mice medulloblastomas (Ptch1+/−model,n=3); Nb, mice neuroblastomas (Th-Mycn model,n=4); lymph, CD8(+) T-cell lymphomas (n=7); mIC, murine intra-cranial tumours (n=5); mE/IC (n=4). (b) Differential subgroups among human tumours were identified by ConsensusClusterPlus R package, as aforementioned. hIC group (human intracranial) consists of 28/28 intracranial tumours and is dissected in three subgroups (hIC1, hIC2 and hIC3). hEC group (human extracranial tumours) consists of 20/22 extracranial tumours and 2/22 intracranial tumours. MB: medulloblastomas, SHH subtype; NB:MYCN-amplified neuroblastomas. (c) AGDEX score performed on each mouse and human subgroups. (d) Left panel: clustering on a set of 540 genes (268+98+42+132) whose higher expression levels specifically define hEC, hIC1, hIC2 and hIC3, respectively; the list is obtained by pair-wise Welcht-test (P≤0.05) analyses, and limited to genes with a fold change |FC|≥1.2 (log2 expression value). Right panel: clustering on the two mouse subgroups using the ortholog genes. Figure 5: Mouse CNS tumours reflect the diversity of human RTs. ( a ) Differential subgroups were identified using ConsensusClusterPlus R package v1.18.0 (with 1,000 resamplings, average linkage hierarchical clustering algorithm and Pearson correlation distance), based on the expressed and variable genes obtained after elimination of background (threshold: 1.2) and invariant genes using RIQR (threshold: 0.75; max(Q3−Q2,Q1−Q 2 )/Q 2 ). Mb, mice medulloblastomas ( Ptch1 +/− model, n =3); Nb, mice neuroblastomas (Th-Mycn model, n =4); lymph, CD8(+) T-cell lymphomas ( n =7); mIC, murine intra-cranial tumours ( n =5); mE/IC ( n =4). ( b ) Differential subgroups among human tumours were identified by ConsensusClusterPlus R package, as aforementioned. hIC group (human intracranial) consists of 28/28 intracranial tumours and is dissected in three subgroups (hIC1, hIC2 and hIC3). hEC group (human extracranial tumours) consists of 20/22 extracranial tumours and 2/22 intracranial tumours. MB: medulloblastomas, SHH subtype; NB: MYCN -amplified neuroblastomas. ( c ) AGDEX score performed on each mouse and human subgroups. ( d ) Left panel: clustering on a set of 540 genes (268+98+42+132) whose higher expression levels specifically define hEC, hIC1, hIC2 and hIC3, respectively; the list is obtained by pair-wise Welch t -test ( P ≤0.05) analyses, and limited to genes with a fold change |FC|≥1.2 (log2 expression value). Right panel: clustering on the two mouse subgroups using the ortholog genes. Full size image Comparisons of mIC and mE/IC, followed by DAVID analyses, revealed that mIC was characterized by a significant over-representation of neuronal development pathways ( Supplementary Data 2 ). In contrast, mE/IC were characterized by few referenced pathways or gene networks. None referred to brain development or neuron differentiation. Comparable diversity in mouse and human tumours The diversity observed within mouse tumours prompted us to investigate whether human RTs also show similar heterogeneity. With this aim, we performed the same three parallel clustering methods on the 50 aforementioned human RTs. In line with the subgroups observed in mouse, unsupervised hierarchical clustering of transcriptome profiles in humans also delineated three subgroups within hIC (hIC1, hIC2 and hIC3, Supplementary Fig. 5a ). NMF ( Supplementary Fig. 5b ) and consensus clustering ( Fig. 5b ; Supplementary Fig. 5c ) both determined that the optimal k value was k =6, also dissecting hIC in the three subgroups identified by hierarchical clustering. Pair-wise differential analyses defined a specific genes signature for each group ( Supplementary Data 3 ). DAVID analysis on these sets of genes confirmed the neuronal pattern for all hIC sub-groups when compared with hEC ( Supplementary Data 3 ); conversely, this latter group was characterized by markers of embryonic morphogenesis and skeletal development. We then further investigated whether mouse tumour subgroups preferentially recapitulate one human group or another, using AGDEX scores. High scores were observed between mIC and hIC2, and mE/IC and hEC ( Fig. 5c ). We then identified lists of genes specifically overexpressed in each human group by pair-wise Welch t -test; clustering mouse tumours on this set of genes also clearly delineated mIC from mE/IC and showed similarities between mIC and hIC2 patterns ( Fig. 5d ). Expression profiles suggest distinct cells of origin The developmental window comprised between E6 and E10 is characterized by the commitment of stem cells to specified progenitors. We therefore postulated that Smarcb1 inactivation at E6-E10 may target such stem or progenitor cells, as cells of origin of the tumours. To get insights in which cells gave rise to which mouse tumours, we correlated transcriptome profiles from our study with transcriptome profiles from stem or progenitor cells from the cephalic region at E6 to E10 in publicly available databases (embryonic Stem Cell (GSE44175), neural progenitor (GSE44175 and GSE44175), neuron (GSE46150), oligodendrocytes derived from neural stem cells (GSE9566), astrocytes derived from neural stem cells (GSE9566), ectomesodermal tissue from the palate (GSE9566) and neural crest (GSE11149)). As shown in Fig. 6a , the highest correlation for mIC was obtained with neuron progenitors, while mE/IC best correlated with ectomesenchyme, a cephalic neural crest cell-derived mesoderm. 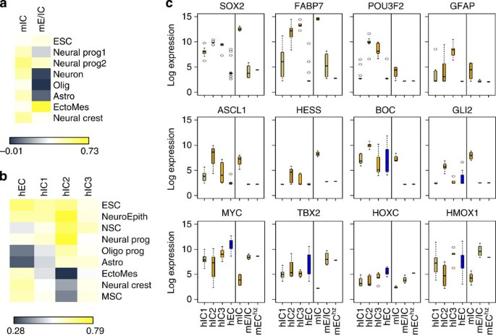Figure 6: Transcriptome profiles suggest various cells of origin for human and miceSMARCB1-deficient tumours. (a) Pearson correlation between transcriptome profiles of mIC and mE/IC from one part, and various mouse embryonal tissues from the other part. ESC: embryonic stem cell (GSE44175). Neural Prog 1, neural progenitor (GSE44175); neural Prog 2, neural progenitor (GSE44175); neuron (GSE46150); olig, oligodendrocytes derived from neural stem cells (GSE9566); astro, astrocytes derived from neural stem cells (GSE9566); EctoMes, ectomesodermal tissue from the palate (GSE9566); neural crest (GSE11149). (b) Pearson correlation between trancriptome profiling of hICs and hEC from one part, and various embryonal tissues from the other part. ESC (GSE55679); NeuroEpith, NeuroEpithelium (GSE55679); NSC, neural stem cell obtained from foetal cortex (GSE15209); neural Prog (GSE56906); glial Prog, glial progenitors (GSE36634); oligo Prog, adult oligodendrocytes progenitors (GSE29368); astro, astrocytes (GSE18959); MSC, mesenchymal stem cells (GSE37603); neural crest (GSE14340); EctoMes (GSE24598). (c) Log2 expression of genes obtained on Affymetrix U133Plus2.0 and MOE430 arrays. Human genes are plotted on the left panels, mouse orthologs on the right panels. hIC1,n=11; hIC2,n=;12 hIC3,n=5; hEC,n=20; mIC,n=5; mE/IC,n=4; mECHzrefers to the face tumour obtained from the heterozygousSmarcb1wt/del_ex1-2model, as a ‘standard’ mouse rhabdoid tumour (n=1). In box plots, the central rectangle spans the first quartile to the third quartile (interquantile range or IQR); the horizontal line inside the rectangle shows the median; whiskers are taken to 1.5 × IQR from the quartile; circles show outliers. For HOXC cluster, the mean expression of all genes in the cluster is plotted as one single value.SOX2,FABP7andPOU3F2are co-expressed in neural stem cells;ASCL1andHES5exert antagonistic effects in neural stem cells to influence the lineage commitment;BOCandGLI2signals the SHH pathway in neural stem cells;TBX2andHMOX1are homeobox genes expressed by mesenchymal cells. Figure 6: Transcriptome profiles suggest various cells of origin for human and mice SMARCB1 -deficient tumours. ( a ) Pearson correlation between transcriptome profiles of mIC and mE/IC from one part, and various mouse embryonal tissues from the other part. ESC: embryonic stem cell (GSE44175). Neural Prog 1, neural progenitor (GSE44175); neural Prog 2, neural progenitor (GSE44175); neuron (GSE46150); olig, oligodendrocytes derived from neural stem cells (GSE9566); astro, astrocytes derived from neural stem cells (GSE9566); EctoMes, ectomesodermal tissue from the palate (GSE9566); neural crest (GSE11149). ( b ) Pearson correlation between trancriptome profiling of hICs and hEC from one part, and various embryonal tissues from the other part. ESC (GSE55679); NeuroEpith, NeuroEpithelium (GSE55679); NSC, neural stem cell obtained from foetal cortex (GSE15209); neural Prog (GSE56906); glial Prog, glial progenitors (GSE36634); oligo Prog, adult oligodendrocytes progenitors (GSE29368); astro, astrocytes (GSE18959); MSC, mesenchymal stem cells (GSE37603); neural crest (GSE14340); EctoMes (GSE24598). ( c ) Log2 expression of genes obtained on Affymetrix U133Plus2.0 and MOE430 arrays. Human genes are plotted on the left panels, mouse orthologs on the right panels. hIC1, n =11; hIC2, n =;12 hIC3, n =5; hEC, n =20; mIC, n =5; mE/IC, n =4; mEC Hz refers to the face tumour obtained from the heterozygous Smarcb1 wt/del_ex1-2 model, as a ‘standard’ mouse rhabdoid tumour ( n =1). In box plots, the central rectangle spans the first quartile to the third quartile (interquantile range or IQR); the horizontal line inside the rectangle shows the median; whiskers are taken to 1.5 × IQR from the quartile; circles show outliers. For HOXC cluster, the mean expression of all genes in the cluster is plotted as one single value. SOX2 , FABP7 and POU3F2 are co-expressed in neural stem cells; ASCL1 and HES5 exert antagonistic effects in neural stem cells to influence the lineage commitment; BOC and GLI2 signals the SHH pathway in neural stem cells; TBX2 and HMOX1 are homeobox genes expressed by mesenchymal cells. Full size image We then similarly compared human tumours with human stem or progenitor cell profiles available in public databases ( Fig. 6b ). The most striking correlation was found between hIC2 and neuro-epithelium, neural stem cells and neuron progenitors; hIC1 and hIC3 showed weaker correlations with these early neuronal lineages. Conversely, high correlation was observed between hEC and embryonic stem cells as well as neural crest-derived cells. To corroborate these correlations based on genome-wide expression, we looked in more detail at the expression pattern of stem or progenitor cell-specific markers, both in mouse and human tumours. hIC2 and mIC were both characterized by the overexpression of SOX2 , POU3F1/2 and ASCL1 , a combination of genes expressed in neural stem cells and capable of reprograming fibroblasts into neurons [19] , [20] ( Fig. 6c , Supplementary Data 2 and 3 ). They also overexpress HES5 , a Notch effector antagonizing the pro-differentiating effects of ASCL1 in neural stem cells at E8-E8.5 (refs 21 , 22 , 23 ), FABP7 , an intracytoplasmic marker of neural stem cells [24] , and components of the SHH pathway ( BOC , GLI2 ) ( Fig. 6c and Supplementary Fig. 6 ). mIC was also characterized by a high expression of Mycn , which was completely absent from mE/IC tumours ( Supplementary Data 2 ). In contrast, hIC1 were characterized by a lower expression of SOX2 and FABP7 , and absence of expression of POU3F2 , ASCL1 , HES5 ( Fig. 6c ; Supplementary Fig. 6 ; Supplementary Data 3 ). However, they strongly expressed OTX2 and ODZ2 , two markers of neural progenitors [25] , [26] ( Supplementary Data 3 ). They also showed higher expression of BMP pathway genes, such as BMP4, BAMBI and SMAD7 ( Supplementary Data 3 ). hIC3 expressed a combination of genes suggesting neural stem cells ( POU3F2 , SOX2 , FABP7 ), but also radial glial ( GFAP ) [27] commitment ( Fig. 6c ; Supplementary Fig. 6 ; Supplementary Data 3 ). All hIC groups showed a high expression of ACTL6A and no expression of ACTL6B , suggesting that these tumours did not yet commit the switch from the ‘neural progenitor’ to the ‘neural’ BAF complex [28] . The same pattern was found in mIC ( Supplementary Fig. 7 ). Finally, hEC showed no expression of these neural genes but overexpressed homeobox genes critically involved in early development of mesodermal-derived structures; among those homeobox genes, TBX2 (ref. 29 ) and HOXA/C genes [30] , [31] ( Fig. 6c ; Supplementary Fig. 6 ) were also found overexpressed in mE/IC. hEC and mE/IC both showed a distinctive expression of TGFB pathway ( TGFBR2 , TGFBR3 , SMAD7 ). Finally, hEC and mE/IC were also characterized by an overexpression of MYC oncogene, which was virtually absent from mIC ( Fig. 6c ). Our data first show that the developmental stage targeted by Smarcb1 inactivation dramatically impacts the type of tumours obtained. Adult mouse tumours in our study are very similar to those published by Roberts et al . [11] . These authors used the Mx-Cre system to drive an inducible inversion of Smarcb1 on interferon or polyI/polyC administration. Our model emphasizes that the occurrence of lymphomas is not due to the Interferon/Mx-Cre system, which might preferentially target liver, spleen or hematopoietic cells [16] . In contrast, the convergence of these two models reveals that T cells are exquisitely sensitive to Smarcb1 deletion in adult mice. Wang et al . [32] showed that a highly specific population of T cells, for example, mature memory CD8(+)CD44 high CD122 low cells, was able to undergo a malignant transformation on Smarcb1- deletion. The absence of these cells in neonates and their expansion throughout life and maturation of the immune system [33] fit with a temporally restricted proneness to developing this type of lymphomas during post-natal life. This lymphoma phenotype is, however, fundamentally different from any SMARCB1 -deficient tumours observed in Humans. Face and neck tumours obtained from heterozygous knockout of Smarcb1 have been suggested to constitute a good mouse model for human extra cerebral RTs. Unfortunately, due to the low penetrance of this model (1/10), we could only include one such tumour in our comparisons of expression profilings. Nevertheless, the co-clustering in a single mE/IC group of the face tumour from the heterozygous model and of intra- and extracranial tumours from our inducible model suggests that the two models lead to similar types of tumours. The assumption that these models recapitulate human extracranial RTs is further corroborated by the high AGDEX correlation obtained between mE/IC and hEC groups. Our highly penetrant, AT/RT-like, mIC group brings major novelties among previously described Smarcb1 -deficient mouse tumours (summarized in Supplementary Table 1 ). Dependent on Smarcb1 inactivation only, they truly mimic human RTs’ oncogenesis. Furthermore, they present strong correlation with hIC2; as such, they now offer a faithful model for at least a subset of AT/RTs. Inactivating Smarcb1 between E6 and E10 provokes a Smarcb1 loss necessarily in embryonic stem cells or progenitors, which are predominant at that time. In the cephalic region at these early developmental stages, the neuroepithelium of the closing neural tube is giving birth to neural stem cells and cephalic neural crest cells. The high correlation between mE/IC and ectomesodermal tissue may suggest cephalic neural crest-derived cells as cells of origin for this group, in consistency with their AGDEX homology with the hEC group, the expression profile of which also correlates with this neural crest cells or MSCs. In contrast, mIC show higher correlation with neural progenitors, which may thus be their cell of origin; this is fully consistent with hIC2 also showing strong correlations with neural stem cells and neural progenitors. Both mIC and hIC2 harbour high levels of SOX2 , ASCL1 , POU3F1/2 and HES5 , genes involved in the fine-tune regulation of neural stem cells commitment in neuronal progenitors. Since the integrity of the SWI/SNF complex is required for the commitment of neuron stem cells into neuronal progenitors [34] , [35] , it may be speculated that targeting Smarcb1 from E6 to E10 in the CNS impairs the progression of neural stem cells through neural differentiation, which may constitute a critical step in oncogenesis. The unexpected heterogeneity within hIC tumours may then reflect that various stem or progenitor cells are able to survive to Smarcb1 inactivation, and subsequently give rise to significantly different tumours. Torchia et al . [36] recently published expression profiling on a series of 51 AT/RT that corroborate our results. They indeed identified a first group of AT/RT that was characterized by higher expressions of ASCL1 and HES5 (NOTCH pathway), FABP7 , POU3F2 , SOX2 and MYCN genes; all those features are reminiscent of our mIC and hIC2 groups and accordingly strongly suggesting a neural origin. In contrast, the second group identified by Torchia et al . was characterized by a higher expression of genes involved in the BMP pathway ( BM4 , BAMBI , SMAD6 ), CLIC6 , OTX2 and MSX1 , all features they describe as ‘mesenchymal’ and which are also characteristic of our hIC1 group. Interestingly, they propose two kinds of cells of origin for AT/RT, one deriving from neural progenitors, and the other having more mesenchymal lineage markers, a conclusion fully consistent with the hypotheses coming from our mouse model. Of note, our study and Torchia’s series both focus on paediatric AT/RT, while a few AT/RT adult cases are reported [37] , challenging the proposed hypotheses of early embryonic progenitors as exclusive cells of origin. One explanation could be that a pool of embryonic neuron stem cells remains until adulthood. Alternatively, one could also hypothesize that adult AT/RT are truly different from their paediatric counterparts, as it was previously published for adult and paediatric medulloblastomas [38] . The observation of neuroglial tumours with BRAF V600E mutation acquiring a AT/RT-like phenotype on SMARCB1 loss [39] illustrates that some cells with abnormal genetic background may tolerate SMARCB1 loss and undergo malignant transformation with a rhabdoid phenotype, without being actual AT/RT, restrictedly defined as an infant disease characterized by a remarkably simple genome. Our results suggest that a restricted early developmental window is required to most efficaciously target the putative pool of cells of origin for AT/RT. Although the lower recombination rate in brain after E10 may influence penetrance, Smarcb1 -deficient cells can be observed at E12 but cannot give rise to tumours. Such an observation is consistent with the lack of tumour phenotype in Smarcb1 flox/flox ;Atoh1-Cre model [40] ; this model demonstrates that Smarcb1 -deficient granule cell precursors fail to develop and lead to severe cerebellum hypoplasia, indicating that AT/RT do not arise from granule cell precursors but from a distinct, developmentally restricted cell population. These important results encourage developing now new conditional Smarcb1 flox/flox mouse models, using Cre ERT2 under the control of promoters specific for each cell type or developmental stage, such as SOX2 (stemness features), ASCL1 (progenitors at the lateral inhibition step), OTX2 (neuronal progenitors) or MSX1 (ectodermal progenitors) to validate our hypothesis. We may then be able to more accurately determine which kind of progenitor can actually tolerate Smarcb1 depletion and give rise to the various AT/RT subgroups. The metabolic failure observed in neonates also exemplifies the time-dependent phenotypes obtained on Smarcb1 loss. The increasing recombination rates during the liver development ( Supplementary Fig. 2a ) as well as the survival of 4/10 neonates when using half doses of tamoxifen ( Fig. 2b ) demonstrated that the variation of phenotypes from E12 to E18 (no death) and after birth (high mortality) might tightly depend on the percentage of remaining Smarcb1 -proficient hepatocytes; presumably also, the maternal liver may supplement a transient foetal liver deficiency until birth. However, the total absence of tumours within the few surviving neonates, neither in the brain nor elsewhere in the body, again argues in favour of a time-restricted phenotype. Neonates may lack both the sufficient pool of neural stem cells to develop AT/RT-like tumours, and the mature memory lymphocytes to develop CD8+ lymphomas. Finally, our model recapitulates the diversity of human RTs in a much broader way than previously published models. In particular, this model offers the first highly penetrant model for intracranial tumours. Interestingly, mIC and hIC2 are both characterized by genes involved in SHH signalling, which is consistent with previous reports linking SMARCB1 loss to GLI1 overexpression [41] . This observation might be of clinical relevance, given the potential sensitivity of some AT/RT cell lines to SHH inhibitors [42] . In that perspective, our model not only brings new insights on the developmental biology underlying RTs oncogenesis; it also offers encouraging conditions for preclinical treatment of this harmful disease. Animals For Smarcb1 flox/flox mouse strain, exons 1 and 2 of Smarcb1 gene were flanked by two loxP sites [13] ; this strain was crossed with a knock-in mouse line harbouring the Cre ERT2 coding region under the control of the Rosa26 locus (Rosa26-Cre ERT2 ) [12] . Mice were genotyped according to these references for Smarcb1 del/flox/wt PCR: forward1: 5′-CTTGCCAGGTGAGCAGTCTG-3′, forward2: 5′-GTTGTTAGTCCCTTTGCTCC-3′, reverse: 5′-GCCACCAGCCAGATGTCATAC-3′. PCR product sizes were: wild-type allele: 150 bp; floxed allele: 250 bp; deleted allele: 400 bp ( Supplementary Fig. 8 ). All experiments were performed on mixed background (129/SV × C57BL/6). The sex ratio within groups was in equilibrium. Protocol and animal housing were in accordance with national regulation and international guidelines [43] . Approval for this study was received from the Institutional CEST review board (Comite d’Evaluation et de Suivi de Recherche Translationnelle) from Curie Institute, and from the Direction Generale de la Recherche et de l’Innovation, Ministere de l’Enseignement Superieur et de la Recherche (authorization number 6,150). We use PGK-Cre mice (from Curie animal facility) to get Smarcb1 wt/del_ex1-2 : Cre is driven by early acting PGK-1 promoter, the recombinase is under dominant maternal control [44] . Smarcb1 wt/del_ex1-2 mice were generated by crossing PGK-Cre female with Smarcb1 flox/wt male. Ten Smarcb1 wt/del_ex1-2 mice (5 males and 5 females, adults) were followed. Smarcb1 del_ex1-2/flox mice were generated by crossing Smarcb1 flox/flox with Smarcb1 wt/del_ex1-2 . The Rosa26-LacZ reporter strain was previously published in Sariono et al . [45] . Tamoxifen administration A single dose of tamoxifen (Sigma, T5648, dissolved at 10 mg ml −1 in sterile ethanol:sun flower oil 1:10) was administrated per os to pregnant Smarcb1 flox/flox ; Rosa26-Cre ERT2 mice at 6, 7, 8, 9, 10, 11, 12, 15 and 18 days post coitum (post-coital plug observation defined day 0) as shown in Supplementary Fig. 3 . All foetuses were delivered by caesarean section (E19) and raised by foster mothers. Neonate (P2 or P3) and adult Smarcb1 flox/flox ;Rosa26-Cre ERT2 mice were injected intraperitoneally with a single conventional dose of tamoxifen (2 mg per 20 g mice). A second cohort of neonates was treated with a single reduced dose of tamoxifen (1 mg per 20 g mice) at P2 ( Supplementary Fig. 3 ). Five to ten Smarcb1 flox/flox ;Rosa26-Cre ERT2 mice were treated with the vehicle (sunflower oil) at all stages of development, in embryos (E6, E9, E12- not later on, since no phenotype was observed in embryos treated with tamoxifen after E12), neonates and adults. R26-Cre ERT2 ; Rosa26-LacZ gestant females were treated with tamoxifen (1 mg per 20 mg) at E6 and E9, LacZ staining was analysed at E15 ( n ≥5 embryos for each point). Histological examination Organs were collected, frozen on dry ice and processed for cryosectionning and macro-dissection) or fixed in AFA (Carlo Erba, ref: 526263001) for histological examination. BAF47 immunohistochemistry was performed on fixed paraffin-embedded tissue using BD, code 612111, clone 25/BAF47, dilution 1/50 (ref. 46 ). CD3 (Dako, code IS503, dilution 1/200), CD4 (Dako, code IS649, clone 4B12, dilution 1/200) and CD8 (Dako, code IS623, clone C8/144B, dilution 1/200) were carried out utilizing commercially staining kit (Dako Envision Kit, K4009 for CD3 and Vector laboratories mouse on mouse basic kit for CD4 and CD8). PAS staining was performed on fixed paraffin-embedded neonate liver as described in ref. 13 . Quantifications were done for PAS by counting the number of positive areas at magnification × 10, in eight livers for 2 mg per 20 g group and six livers for 1 mg per 20 g group. Frozen sagittal section β-galactosidase stainings ( Supplementary Fig. 2 ) were performed as described in Echelard et al . [47] , on embryos freshly taken out (E6, E9, E12) at E15 and on neonates. Mouse tumours macrodissection and RNA extraction Frozen brains were serially sectioned using a cryostat at 4 μm; quick Hematoxilin stainings were performed on each section until a tumour could be identified; macrodissection was then performed with a sterile scalpel. Small pieces of tissue containing the tumour cells were frozen at −80 °C until RNA preparation. The tumour RNAs were extracted using a miRNeasy mini kit (Qiagen ref: 217004). Human samples selection and RNA extraction Human RTs were referred to our Institute for assessment of SMARCB1 gene status. We selected tumours only when the diagnosis was made before 5 years of age. BAF47 immunohistochemistry was assessed as described in ref. 46 and SMARCB1 molecular analysis was performed as described in ref. 48 . Samples were used for research purposes according to French Huriet Law regarding research on human tissues. Total RNAs were obtained from frozen samples using Qiagen QIAamp RNAeasy kit, according to the manufacturer’s procedures. The tumour cell content was visually estimated before RNA extractions; tumour cell content lower than 60% was an exclusion criteria. Samples were used according to the French Hurriet law (88–1,138) regarding research on human tissues. Frozen samples were provided by French tumour banks from consenting patients. Approval for this study was received from the Institutional CEST review board (Comite d’Evaluation et de Suivi de recherche Translationnelle) form Curie Institute. Quantitative RT-PCR Reverse transcription was carried out on 0.5 μg total RNA from human and mouse tumours with oligo(dT) primers following the manufacturer’s instructions (High capacity cDNA Reverse Transcription Kit, Applied Biosystems). Expression levels of genes were analysed using real-time, quantitative PCR. All amplifications were done using the SYBR Green PCR Master Mix (Applied Biosystems) and the CFX384 machine (Bio-Rad). The relative quantification for gene expression was determined using the 2 −ΔΔCt method. The TBP gene was used as internal control for data normalization. Primers used in this publication are available in Supplementary Table 2 . Microarray analysis Micro-array data have been deposited in the GEO database under accession code GSE64019. In Smarcb1 flox/flox ;Rosa26-Cre ERT2 mice, transcriptomes of seven Smarcb1 -deficient lymphomas, nine Smarcb 1-deficient intracranial tumours and one soft-tissue tumour were analysed. From the Smarcb1 delx_ex2/wt mouse model, only one face tumour was analysed. The transcriptomes of seven Ctnnb del_ex3 lymphomas (GSE7050), three neuroblastomas (previously published, GSE46583) [14] and four medulloblastomas were analysed. In humans, 20 extra-CNS RTs, 30 intra-CNS RTs, 8 SHH medulloblastomas and 8 MYCN amplified neuroblastomas were profiled. cDNA from murine tumours were hybridized to Affymetrix Murine MOE430 2.0 arrays, while human samples were hybridized to Affymetrix U133Plus2.0 arrays. Gene expression data was normalized using gcRMA algorithm on custom Brainarray CDF [49] . Differential subgroups were defined using different methods: unsupervised hierarchical clustering (average linkage and Pearson correlation distance), consensus clustering (using ConsensusClusterPlus R package v1.18.0, with 1,000 resamplings, average linkage hierarchical clustering and Pearson correlation) and NMF (using NMF R package, with standard NMF algorithm method performed on 30 runs). The optimal number of subgroups have been defined on the lower proportion of ambiguous clustering value (PAC k = CDF k (valueindex(max))−CDF k (valueindex(min))) and biological knowledge for consensus clustering method; and on the better cophenetic correlation score and biological knowledge for NMF method. All these methods are based on the expressed and variable genes obtained after elimination of background (threshold: 1.2) and invariant genes using RIQR (threshold: 0.75; max(Q3−Q2,Q1−Q3)/Q2). Differentially expressed genes between two groups were defined using Welch t -test ( P ≤0.05 adjusted with Benjamini and Hochberg) and fold change (|FC|≥1.2). Concordance of orthologous genes between human and mouse was made with HomoloGene. For intraspecies comparisons, Pearson correlation score on transcriptome profilings were calculated by correlating the means of each gene expression value, after filtering those below the background and unvariant genes. The agreement between human and mouse gene expression tissues was evaluated using AGDEX (Agreement of differential expression) R package v.1.6.0, based on a statistical procedure described in Johnson et al . [18] . The reference tissues were prefrontal cortex—downloaded from the GEO database (GSE11512 for human, GSE16660 for mice). Comparisons between human MYCN -amplified neuroblastomas (previously published, GSE12460) and murine neuroblastomas from the Th-Mycn model (previously published, GSE46583) on one hand, and SHH medulloblastomas in humans [50] (previously published, GSE12992) and shh medulloblastomas from Ptch1 +/− models, on the other hand, served as controls. All bioinformatic analyses were performed with R software environment. Accession codes: The micro-array data have been deposited in the GEO database under accession code GSE64019 . How to cite this article: Han, Z.-Y. et al . The occurrence of intracranial rhabdoid tumours in mice depends on temporal control of Smarcb1 inactivation. Nat. Commun. 7:10421 doi: 10.1038/ncomms10421 (2016).